Female song is widespread and ancestral in songbirds Bird song has historically been considered an almost exclusively male trait, an observation fundamental to the formulation of Darwin’s theory of sexual selection. Like other male ornaments, song is used by male songbirds to attract females and compete with rivals. Thus, bird song has become a textbook example of the power of sexual selection to lead to extreme neurological and behavioural sex differences. Here we present an extensive survey and ancestral state reconstruction of female song across songbirds showing that female song is present in 71% of surveyed species including 32 families, and that females sang in the common ancestor of modern songbirds. Our results reverse classical assumptions about the evolution of song and sex differences in birds. The challenge now is to identify whether sexual selection alone or broader processes, such as social or natural selection, best explain the evolution of elaborate traits in both sexes. The evolution of elaborate traits has almost universally been attributed to sexual selection acting on males [1] , [2] , [3] . Elaborate signal traits in females are often phenotypically similar to those of males, but there is controversy over whether they arise similarly through sexual selection, or through broader processes such as social or natural selection [4] , [5] , [6] , [7] . Resolution of this debate is constrained by a paucity of knowledge about female signal traits [1] , [3] , a bias that is particularly pronounced in the study of bird song [8] , [9] . The majority of bird song research has been conducted under the premise that songbirds (oscine passerines) have evolved complex song and large repertoires through sexual selection on males via male–male competition and female choice [10] , [11] . In this scenario, Darwin himself suggests that the primary role of females is to listen: ‘... female birds, by selecting, during thousands of generations, the most melodious or beautiful males, according to their standard of beauty, might produce a marked effect’ [12] . Instances of female song have traditionally been dismissed as rare, atypical or the outcome of hormonal aberrations [13] , [14] , [15] . However, a number of studies have proposed that this view is erroneous [8] , [9] , [16] , and reflects a geographical bias towards temperate North America and Europe, where species with male-only song are disproportionately common compared with other biogeographical regions [17] , [18] , [19] . While there is growing acknowledgement that female song is more common and evolutionarily important than previously thought [9] , [18] , [20] , this has not been assessed quantitatively across both phylogenetically and geographically diverse lineages [16] , [21] , [22] . Here we propose and test an evolutionary scenario that is radically different from the framework used since Darwin applied his theory of sexual selection to bird song: rather than being rare and atypical, we propose that female song is widespread and ancestral in songbirds. We base this hypothesis on two observations [9] . First, the majority of songbird biodiversity exists in tropical regions [23] , where both females and males of many species sing [17] , [18] , [20] . Second, female song is widespread in Australasia [19] , the region from which songbirds are thought to have originated [24] . To provide a quantitative test of this hypothesis, we first surveyed the occurrence of female song, and then used ancestral state reconstruction to examine the likelihood that females sang in the ancestor of all songbirds. We focused on the songbirds (oscine passerines) because they are the major radiation of birds known for learned, sexually selected, complex songs [15] . We included all families of songbirds except those belonging to the most recent radiation, the Passerida [24] . We omitted the Passerida because they are so nested within the songbird phylogeny that they contribute only 0.08% to reconstruction of the ancestral node in songbirds (although they are the most specious Parvorder of songbirds with 3,822 of 5,023 songbird species [25] ). This resulted in our survey including 44 of ~112 songbird families [25] . We show that female song occurs in over two-thirds of surveyed songbird species and families. Moreover, ancestral state reconstruction reveals that females sang in the ancestral songbird, a result that challenges the view that sexual dimorphism in song production arises primarily as a result of sexual selection. Prevalence of female song We investigated the presence of female song in 1,141 songbird species. 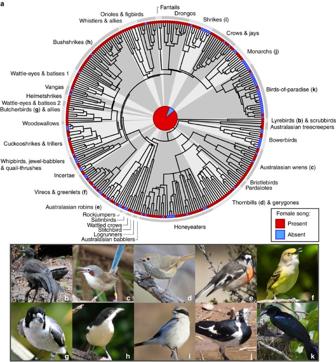Figure 1: Ancestral state reconstruction of female song on a phylogenetic tree of the oscine passerines. The tree (a) includes all species for which we could unambiguously score female song as present or absent (323/1,141 species from 34/44 songbird families). Female song was present in 229 species (32 families; red terminal nodes) and female song was absent in 94 species (19 families; blue terminal nodes). The pie chart in the centre shows that female song is reconstructed as present (red) in the common ancestor of modern songbirds (92% maximum-likelihood probability strongly supported by a likelihood decision threshold of 2.0). Pictures show females of the following species with female song from families throughout the phylogeny; (b) superb lyrebird (Menura novaehollandiae;figure reproduced with permission from V. Dunis), (c) purple-crowned fairywren (Malurus coronatus; figure reproduced with permission from M. Hall), (d) brown thornbill (Acanthiza pusilla; figure reproduced with permission from J.J. Harrison), (e) scarlet robin (Petroica boodang; figure reproduced with permission from K. Odom), (f) white-eyed vireo (Vireo griseus; figure reproduced with permission from F. Jacobsen), (g) grey butcherbird (Cracticus torquatus; figure reproduced with permission from A. Kearns), (h) tropical boubou (Laniarius aethiopicus; figure reproduced with permission from J. Friedman), (i) loggerhead shrike (Lanius ludovicianus; figure reproduced with permission from F. Jacobsen), (j) magpie-lark (Grallina cyanoleuca; figure reproduced with permission from M. Hall), (k) curl-crested manucode (Manucodia comrii; figure reproduced with permission from T. Laman). Using stringent criteria (see Methods), we were able to score 323 species (representing 34 of the 44 songbird families examined, see Supplementary Table 1 ) for the presence or absence of female song based on several major sources (primarily Handbook of the Birds of the World [26] , see Methods for complete list). Our survey showed that female song is present in 71% of the songbird species in our sample (229 of 323 species), including 32 of 34 oscine families that had information on which sexes sing ( Fig. 1 , Supplementary Table 1 ). This result is complemented by a regional study that found female song in 43% of European passerine species, primarily Passerida (23 out of 26 families) [21] . Together with our worldwide survey, which included information from an additional 34 songbird families, there is strong evidence that female song is globally and phylogenetically widespread. Figure 1: Ancestral state reconstruction of female song on a phylogenetic tree of the oscine passerines. The tree ( a ) includes all species for which we could unambiguously score female song as present or absent (323/1,141 species from 34/44 songbird families). Female song was present in 229 species (32 families; red terminal nodes) and female song was absent in 94 species (19 families; blue terminal nodes). The pie chart in the centre shows that female song is reconstructed as present (red) in the common ancestor of modern songbirds (92% maximum-likelihood probability strongly supported by a likelihood decision threshold of 2.0). Pictures show females of the following species with female song from families throughout the phylogeny; ( b ) superb lyrebird ( Menura novaehollandiae; figure reproduced with permission from V. Dunis), ( c ) purple-crowned fairywren ( Malurus coronatus ; figure reproduced with permission from M. Hall), ( d ) brown thornbill ( Acanthiza pusilla ; figure reproduced with permission from J.J. Harrison), ( e ) scarlet robin ( Petroica boodang ; figure reproduced with permission from K. Odom), ( f ) white-eyed vireo ( Vireo griseus ; figure reproduced with permission from F. Jacobsen), ( g ) grey butcherbird ( Cracticus torquatus ; figure reproduced with permission from A. Kearns), ( h ) tropical boubou ( Laniarius aethiopicus ; figure reproduced with permission from J. Friedman), ( i ) loggerhead shrike ( Lanius ludovicianus ; figure reproduced with permission from F. Jacobsen), ( j ) magpie-lark ( Grallina cyanoleuca ; figure reproduced with permission from M. Hall), ( k ) curl-crested manucode ( Manucodia comrii ; figure reproduced with permission from T. Laman). Full size image Ancestral state reconstruction We mapped the data from our survey of female song onto a recent and exhaustive phylogenetic tree for the passerines constructed from a supermatrix containing all available GenBank gene sequences (covering 66.5% of passerine species) [27] . This provided estimates of actual branch lengths and species relationships, important for maximum-likelihood ancestral state reconstruction. We reconstructed the ancestral state for the oscines using both parsimony (unordered) and maximum-likelihood (Markov k-state one-parameter, Mk1, and asymmetrical two-parameter Markov k-state, Asymm.2) analyses in Mesquite v2.75 (ref. 28 ) ( Table 1 ). All three models agreed that female song was more likely to be present than absent in the ancestor of songbirds ( Table 1 ). Parsimony analysis unequivocally (100% probability) reconstructed female song as the ancestral state, and maximum likelihood indicated a 91.9% probability that females sang in the ancestor of the oscine passerines (strongly supported by a likelihood decision threshold of 2.0; Fig. 1 , Table 1 ). Additional reconstructions using a sample of 100 molecular trees from Jetz et al. [29] gave nearly identical results for both parsimony (100%) and maximum likelihood (92.6%). Table 1 Multiple ancestral state reconstructions of female song in oscine passerines. Full size table This finding was robust to missing data arising from excluding the Passerida and incomplete information. First, we tested the effect of the Passerida on the probability that female song was present in the ancestor by scoring all members as ‘female song present’ (which gave a 93% probability that female song is ancestral) and then all members as ‘female song absent’ (85% probability, Table 1 ). The conclusion that song in females is ancestral is thus robust, even under the most conservative assumption that no single Passerida species has female song, which is empirically unfounded [8] , [21] . Second, to assess the impact of species with no information on female song, we conducted sensitivity analyses. We randomly assigned these taxa different proportions of scores of ‘female song present’ and ‘female song absent’ ( Table 1 ). Our result was robust to randomly scoring female song as absent in two-thirds of species with no information on female song (87% probability, Table 1 ). This is a conservative estimate, since we found female song to be absent in less than one-third of species with information on female song. Our finding that song is both widespread and ancestral in female songbirds calls for a re-evaluation of the pervasive view of bird song as an epigamic male trait that has evolved through sexual selection [8] . Females, as well as males, can experience intense competition over ecological resources, which may select for traits that signal their competitive prowess or ownership of resources [5] . Since song originally evolved in both sexes, this broader conceptual framework of social selection, in which sexual selection is one component of selection resulting from social interactions [4] , [7] , may be useful for studying the evolution and maintenance of song in both males and females. Moreover, our results show that the current sexual dimorphism in song seen in some species reflects recent evolutionary losses of female song from an ancestor that had both male and female song ( Fig. 1 ). Song in both sexes in the ancestor to the modern songbirds suggests that the current sexual dimorphism in elaborate traits results from selection against these traits in females, paralleling recent findings on the evolution of plumage dichromatism in some birds [16] , [30] , [31] . This perspective prompts the question of why females have lost song secondarily in certain lineages. Four correlates of female song have been identified: a tropical distribution [18] , year-round territoriality [19] , convergent sex roles [20] and sexual dichromatism in carotenoid-based colours [21] . Correspondingly, phylogenetic analysis of New World blackbirds showed loss of female song was correlated with loss of a composite life-history pattern of monogamy, dispersed nesting (a proxy for territoriality) and non-migratory behaviour [16] , [32] . Migration is also associated with more elaborate song and higher testosterone levels in males [21] , [33] , suggesting that the evolution of migration might be an important driver of sex role divergence and sexual dimorphism in song. This and related hypotheses could be tested in future comparative analyses in the range of taxa that have lost female song, and in songbirds in general. Sex differences in the developmental neuroanatomy of songbirds are also consistent with an early origin of bird song in both sexes. Male and female songbirds develop equivalent neural song production systems during embryonic development [34] . The song nuclei subsequently atrophy in females of species that lack female song altogether [35] . Exposure of these females to steroid hormones as juveniles can induce masculinization of brain morphology and functional capacity for song [36] . Thus, the widely studied sexual dimorphism in the song control system of some songbirds, like sexual dimorphism in song production itself [37] , is consistent with secondary loss of these attributes in females of some species. Greater variation in the expression of song and higher rates of song loss in females than in males suggest that female songbirds would provide an ideal model for comparative studies investigating candidate genes and molecular pathways regulating song control and vocal learning in birds [38] , [39] . In light of our results, female song can no longer be considered an evolutionary oddity. Rather, song in females is phylogenetically widespread and ancestral in songbirds. The exciting challenges now are to identify the mechanisms that mediate the striking diversity and plasticity seen in the modern-day songbird brain and behaviour as well as the selection pressures driving the maintenance, elaboration and loss of female song in nature. Female song data set We gathered information on female song for every oscine passerine species listed in Sibley and Monroe [40] for all oscine families except members of the Passerida [24] . We did not score Passerida because they are the most recent radiation within the oscines [24] and therefore contribute the least quantitatively to ancestral state reconstruction. In ancestral state reconstruction, divergences closest to the ancestral node have the greatest weight on the ancestral state. Based on parsimony, we calculated that although the Passerida contain ~3,822 species [25] , they are the most recent radiation within songbirds; therefore, they contribute <1/1,280 (0.08%) to reconstruction of the ancestral node of the oscine passerines. However, we did test the impact of different scorings of Passerida on the overall result (see Ancestral state reconstruction section of Methods). In addition to species listed in Sibley and Monroe [40] , we also scored species found in the Hugall and Stuart-Fox [27] passerine tree that were not recognized by Sibley and Monroe [40] . In total, we investigated the presence and absence of female song in 1,141 oscine species using several major sources of species accounts [26] , [41] , [42] , [43] , [44] , [45] , [46] , [47] , [48] , [49] , [50] . Scoring the prevalence of female song We gave all of the above species one of four scores based on documentation of their vocal behaviour: P=female song present, A=female song absent, N=no species-specific song or U=unknown. We scored species as having female song (P) when females were specifically described as having song, pair members perform synchronized or antiphonal duets, or both pair members or all group members sing together. We were particularly careful, especially in the last instance, to assign female song only when the vocalization used to make the assignment was referred to as song (for example, we did not use descriptions of chorusing or general group vocalizing to establish female song because females may use calls rather than songs in these contexts). We scored female song as absent (A) when the account specifically stated that song was only by males, or when song was described as a characteristic of males (for example, males sing) and female vocalizations were described as simple calls. We scored species as having no song (N) if all the vocalizations for that species were described as calls and were broadband or simple (that is, 1–2 syllable) sounds, or if the species account directly stated that the species does not have song (such species regularly included members of the ravens, jays, crows and other social corvoidea). Species were scored as unknown (U) if there was not enough song information to make another designation. This included species for which there was no information on which sex produces songs, or if it was unclear whether the species sang at all. Song was reported without mention of the sex of the singer in 678 of the 1,141 species scored (59.4%). Many of these cases were monochromatic species from the Asia-Pacific region and other (primarily tropical) poorly studied geographic regions. Based on our criteria and the documentation of sex-specific song, we were able to score presence or absence of female song unequivocally for 323 species. Supplementary Table 1 provides totals for final scoring by family and Supplementary Fig. 1 shows species scored as female song present versus absent on the phylogenetic tree. The data gathered on female song for all species surveyed have been deposited online at Dryad (http://datadryad.org/), under data identifier doi:10.5061/dryad.0sd41. Phylogenetic trees used To reconstruct female song, we overlaid our character scores on the passerine tree by Hugall and Stuart-Fox [27] . Their tree was constructed from a supermatrix containing 66.5% of all passerine species (nomenclature following IOC 2.4 species [27] , [51] ), including all available genetic data in GenBank at the time of publication. The tree therefore contained calibrated branch lengths based on molecular divergence, important for maximum-likelihood reconstruction [27] . Branch lengths were calibrated using a relaxed-clock with an arbitrary mean rate of 0.01 (ref. 27) [27] . The Hugall and Stuart-Fox [27] tree represents the most comprehensive tree for species in our study, so was ideal for our purposes. To be certain that our results were not dependent on any one topology, however, we also analysed our data using 100 randomly sampled trees from Jetz et al. [29] (we used their molecular tree with the Hackett backbone). The taxa in the two trees were comparable; however, 80 species in our survey and the tree by Hugall and Stuart-Fox [27] were not in the tree by Jetz et al. [29] The results of analyses using trees by both Jetz et al. [29] and Hugall and Stuart-Fox [27] were nearly identical: all trees reconstructed female song as the ancestral state using parsimony (100% for all trees) both excluding Passerida and when all Passerida were scored as female song absent and present. For our main analysis excluding Passerida, Mk1 maximum likelihood revealed a 92.6% likelihood that female song was ancestral using the Jetz et al. [29] tree and a 91.9% likelihood using the Hugall and Stuart-Fox [27] tree. When female song was scored as absent for all Passerida, we found a 85.9% likelihood that female song was ancestral using the trees by Jetz et al. [29] and a 84.8% likelihood using the Hugall and Stuart-Fox [27] tree. Finally, when all Passerida were scored as female song present, the trees by Jetz et al. [29] revealed a 92.9% likelihood that female song was ancestral, whereas the tree by Hugall and Stuart-Fox [27] revealed a 92.6% likelihood. These results show that our findings are robust to tree topology. The Hugall and Stuart-Fox [27] tree contained 281 of the 323 species for which we had song information, with those species not included in the tree distributed across 17 of the 32 families with female song information, and 90% had female song; therefore, we are confident that their exclusion did not bias our ancestral state reconstruction towards female song. We then removed species that were scored as having no song. We pruned the tree to create three trees with slightly different taxa for subsequent analyses. The tree for our main analysis of whether female song was ancestral included species scored as P (present) and A (absent) and excluded those scored as N (no song) and U (unknown). To assess the impact of missing information, we also prepared a tree containing species scored as female song present or absent (categories P and A) plus Passerida, and another tree containing species scored as female song present or absent plus species scored as unknown (categories P, A and U). Ancestral state reconstruction To determine the most likely ancestral state of female song, we ran three ancestral-state reconstruction models and compared their overall agreement—a well-accepted method for inferring confidence in a reconstruction [45] . We first used unordered parsimony and Markov k-state one-parameter (Mk1) maximum-likelihood reconstructions in Mesquite v2.75 (ref. 28 ). Both models assume equal rates of change between character states. Maximum likelihood provides a good comparison to parsimony because it takes into account the amount of divergence between species (represented by branch lengths) and estimates the uncertainty associated with character reconstruction. We also ran an asymmetrical two-parameter Markov k-state maximum-likelihood model (Assym.2) to test the robustness of our results to departures from the assumption of equal rates of gains and losses of male and female song. We have no a priori reason to believe that gains of female song are more or less costly than gains of male song; therefore, we believe a model with equal rates is likely the most informative [52] . Nevertheless, all models returned high probability and therefore agreed that female song was ancestral ( Table 1 ). To test the robustness of the reconstruction to the uncertainty of missing data, we ran two additional analyses. To examine the impact of Passerida, we ran Mk1 maximum-likelihood models on the tree containing species with female song present or absent plus all Passerida. We ran models for Passerida scored in one of two ways: either as all ‘female song present’ or as all ‘female song absent’. For both models, we used a rate of 0.025 to reconstruct the ancestral state. We used this constant rate of evolution because different proportions of female song drastically altered the rate of evolution calculated for the reconstructions, preventing accurate estimation of ancestral states (for example, allowing the model to specify its own rate-inflated reconstruction for both scenarios to a 99% likelihood that female song was ancestral). The rate of 0.025 was calculated based on the reconstruction that included only species with clear, sex-specific song information. Neither reconstruction differed substantially from the reconstructions without the Passerida ( Table 1 ). To examine the impact of species without sex-specific song information, we randomly assigned different proportions of female song to species scored as unknown. We assigned these species proportions of ‘female song absent’ equal to, twice as common and four times as common as ‘female song present’, as well as scoring all these species as ‘female song absent’. We used a maximum-likelihood Mk1 model with the constant rate of 0.025, as mentioned above. In order for the absence of female song to be a more likely ancestral state, species without female song (absent) would need to be five times more common than species with female song (present). Given that species with female song were twice as common as species without female song in species with sex-specific song information, this scenario seems unlikely ( Table 1 ). How to cite this article: Odom, K. J. et al. Female song is widespread and ancestral in songbirds. Nat. Commun. 5:3379 doi: 10.1038/ncomms4379 (2014).